A genome-wide regulatory network identifies key transcription factors for memory CD8+T-cell development Memory CD8 + T-cell development is defined by the expression of a specific set of memory signature genes. Despite recent progress, many components of the transcriptional control of memory CD8 + T-cell development are still unknown. To identify transcription factors and their interactions in memory CD8 + T-cell development, we construct a genome-wide regulatory network and apply it to identify key transcription factors that regulate memory signature genes. Most of the known transcription factors having a role in memory CD8 + T-cell development are rediscovered and about a dozen new ones are also identified. Sox4 , Bhlhe40 , Bach2 and Runx2 are experimentally verified, and Bach2 is further shown to promote both development and recall proliferation of memory CD8 + T cells through Prdm1 and Id3 . Gene perturbation study identifies the interactions between the transcription factors, with Sox4 positioned as a hub. The identified transcription factors and insights into their interactions should facilitate further dissection of molecular mechanisms underlying memory CD8 + T-cell development. Immunological memory refers to faster and stronger responses to re-encounter of the same antigen. The basis for this enhanced response is the persistence of more abundant and intrinsically more reactive antigen-specific memory T and B lymphocytes that are generated following the initial antigen stimulation. Memory CD8 + T cells are usually generated following antigen-stimulated T-cell activation and expansion. In a typical CD8 + T-cell response, naive CD8 + T cells are activated to undergo clonal expansion when stimulated by appropriate antigen [1] . The resulting T cells acquire effector functions and migratory properties that allow them to clear antigens in both lymphoid and non-lymphoid organs. As antigen is cleared, most of the effector T cells die by apoptosis and only a small fraction survive and differentiate into memory CD8 + T cells. Memory CD8 + T cells are often divided into two subsets. Effector memory T cells (T EM ) are CD62L lo CCR7 lo and capable of rapid expression of effector functions following antigen stimulation to confer faster memory response. Central memory T cells (T CM ) are CD62L hi CCR7 hi and proliferate extensively upon antigen restimulation to confer stronger memory response. Memory CD8 + T cells are developmentally programmed as they express a specific set of memory signature genes (MSGs) [2] , [3] , which confer them with characteristic memory phenotype and function. Like many developmental processes, memory CD8 + T-cell development is ultimately controlled by transcription factors (TFs) that integrate external and internal signals to regulate the expression of the MSGs. In recent years, several studies have shed light on TFs that regulate the development of memory CD8 + T cells. T-bet (encoded by Tbx21 ) and Eomesodermin (encoded by Eomes ), both member of the T-box family, are essential for the differentiation of effector and memory CD8 + T cells [4] , [5] , [6] . Tcf7 is a TF downstream of the Wnt signalling. Consistent with the observation that activation of Wnt/β-catenin signalling promotes memory CD8 + T-cell development by suppressing terminal differentiation of effector T cells [7] , [8] , Tcf7-deficiency in CD8 + T cells impairs T CM differentiation [9] . Klf2 has been shown to be associated with memory CD8 + T-cell development [10] probably by directly controlling the expression of cell surface receptors S1P1 and CD62L [11] , [12] . Id2 and Id3 , the E-box-containing transcription suppressors, appear to regulate the development of memory CD8 + T-cell subsets [13] . Id2-knockout mice are deficient in memory CD8 + T cells, but effector T cells generated in these mice are CD127 hi CD62L hi , a phenotype similar to T CM [14] . Deficiency in Id3 inhibits, whereas overexpression of Id3 promotes memory CD8 + T-cell development [15] . The B-cell transcriptional repressor Blimp-1 (encoded by Prdm1 ) promotes the terminal differentiation of effector CD8 + T cells and is required for recall response of memory T cells [16] , [17] . Despite these progresses, the current understanding of transcriptional regulation of memory CD8 + T-cell development is still limited, as additional TFs as well as their coordination are likely required to respond to external and internal signals in order to establish the MSG programme for memory CD8 + T-cell development. In this study, we assemble a genome-wide regulatory network associated with the development of CD8 + T cells using publicly available gene expression data and a reverse-engineering algorithm. This regulatory network is applied to identify key TFs that regulate memory CD8 + T-cell development using the master regulator analysis (MRA) of the MSGs of CD8 + T cells. The inferred TFs include most of the known TFs as well as a dozen new TFs with limited functional information in CD8 + T-cell differentiation. A regulatory module controlling the MSGs is constructed and the high accuracy of the regulations in the module is verified using ChIP-PCR. Gene perturbations identify multiple regulatory motifs among the key TFs, suggesting their complex regulations during the memory CD8 + T-cell development. Four of the newly identified key TFs ( Sox4 , Bhlhe40 , Bach2 and Runx2 ) are experimentally validated to regulate memory CD8 + T-cell development and function. Bach2 is shown to promote memory CD8 + T-cell development and recall proliferation through Id3 and Prdm1. Our study represents the most comprehensive analysis of TFs and their interactions in memory CD8 + T-cell development to date. The identified TFs and the insights into their mode of interactions provide a foundation for further dissecting the molecular mechanisms underlying memory CD8 + T-cell development. Identification of TFs associated with memory CD8 + T cells We collected 386 gene expression profiles of naive, effector and memory CD8 + T cells of the mouse from 35 independent GEO data sets ( Supplementary Table S1 ). A total of 1,445 genes coding putative TFs [18] were manually mapped to the latest mouse genome to eliminate redundant and erroneous annotations, resulting in a total of 1,038 putative TFs. Among these putative TFs, 464 were expressed during the naive to effector to memory CD8 + T-cell development (see Methods for detail). Using a reverse-engineering algorithm CLR (context likelihood of relatedness) [19] , the 386 gene expression profiles and the 1,038 putative TFs, a genome-wide regulatory network was assembled. The network consisted of 107,157 interactions among 11,032 genes. In all, 62,272 interactions (58%) were between the 276 of the 464 expressed putative TFs and 8,572 target genes, suggesting that interactions are enriched among the expressed genes ( P <0.001, binomial test). Furthermore, 3,219 of these interactions involve 154 out of 196 (79%) identified MSGs [3] ( Supplementary Fig. S1 ). To identify key TFs that regulate MSGs, we applied the MRA to the CLR-inferred interactions ( Fig. 1a , see Methods). The MRA algorithm computes the statistical significance of overlaps of all interactions of each TF (inferred by CLR) with MSGs or a control gene set by a binomial test. From the 1,038 putative TFs, MRA identified 60 MSG-specific TFs at P <0.05 (binomial test), all of which are expressed in CD8 + T cells ( Supplementary Table S2 ). These 60 candidates were filtered by removing those whose knockout does not have any immune system phenotype as defined in MGI (Mouse Genome Informatics) [20] . The positive candidates were then analysed for enrichment of DNA-binding motifs among MSGs or differential expression among naive, effector and memory CD8 + T cells (see Methods). 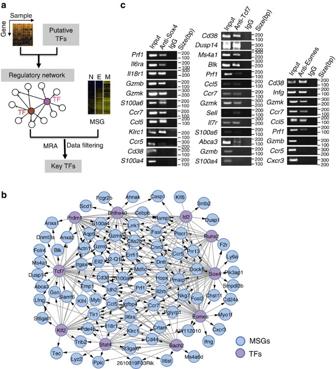Figure 1:Construction of regulatory network of memory CD8+T cells. (a) Schematic diagram of regulatory network analysis for identifying key TFs. N, E, and M, naive, effector and memory CD8+T cells, respectively. (b) The regulatory module of the top 10 TFs (orchid circles) and their MSGs (blue). (c) ChIP-PCR analysis of Sox4, Tcf7 and Emoes-regulated MSGs. ChIP was carried out with CD8+T cells expressing the 2C TCR using antibodies specific for Sox4, Tcf7 or Eomes or control IgG antibodies. Promoter regions of the indicted genes were amplified using the precipitated DNA. Shown are PCR products after electrophoresis. This led to 21 key TFs that were ranked according to the numbers of MSG they regulate ( Table 1 ). Text-mining of public references on these 21 TFs revealed that 8 of 12 known TFs, which have been reported to be involved in memory CD8 + T-cell development and function [21] , [22] , [23] , [24] , were identified by our analysis. These results show that our systematic approach is valid for identifying TFs that regulate memory CD8 + T-cell development. Figure 1: Construction of regulatory network of memory CD8 + T cells . ( a ) Schematic diagram of regulatory network analysis for identifying key TFs. N, E, and M, naive, effector and memory CD8 + T cells, respectively. ( b ) The regulatory module of the top 10 TFs (orchid circles) and their MSGs (blue). ( c ) ChIP-PCR analysis of Sox4, Tcf7 and Emoes-regulated MSGs. ChIP was carried out with CD8 + T cells expressing the 2C TCR using antibodies specific for Sox4, Tcf7 or Eomes or control IgG antibodies. Promoter regions of the indicted genes were amplified using the precipitated DNA. Shown are PCR products after electrophoresis. Full size image Table 1 Ranking of the 21 key TFs identified by master regulator analysis. Full size table Validation of a regulatory module for MSGs To further explore the relative importance of the 21 identified TFs in regulating MSGs, we constructed a regulatory module using the top 10-ranked TFs ( Fig. 1b ). The resulting module contained 56% (86 out of 154) of MSGs that were present in the entire network ( Supplementary Fig. S1 ). To verify this regulatory module, chromatin immunoprecipitation (ChIP) was performed for the top three TFs, Sox4 , Tcf7 and Eomes , in CD8 + T cells followed by PCR amplification of promoter regions (within 1 kb upstream of the transcription-starting site) of randomly selected MSGs that were predicted to be regulated by Sox4 or Tcf7 or Eomes . As shown in Fig.1c,d ( Supplementary Fig. S15 ), promoter regions of 10 out of the 12 randomly selected Sox4 -regulated MSGs were amplified. Similarly, 12 out of 14 randomly selected Tcf7 -regulated MSGs and 6 out of 9 randomly selected Eomes-regulated MSGs were amplified. 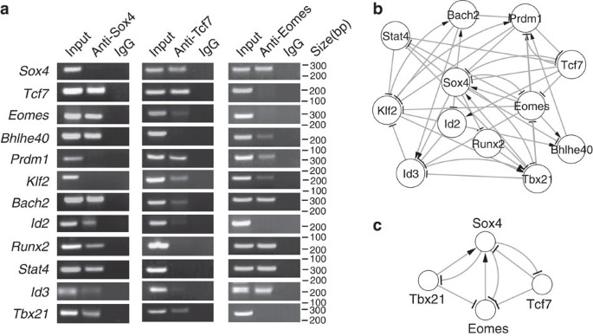Figure 2:Construction of perturbation network of TFs in CD8+T cells. (a) ChIP-PCR analysis. ChIP was carried out with 2C T cells using antibodies specific for Sox4, Tcf7 or Eomes or control IgG antibodies. Promoter regions of the indicted genes were then amplified using the precipitated DNA. Shown are PCR products after electrophoresis. (b) Perturbation network based onTable 3. (c) An example of network motifs from the perturbation network. On average, 80% of the tested promoter regions were immunoprecipitated with antibodies specific for each of the three TFs ( Table 2 ), confirming the high accuracy of the constructed regulatory module. Furthermore, when the cumulative coverage of MSGs was plotted as a function of each of the 21 TFs, the top two TFs, Sox4 and Tcf7 , were shown to regulate 42% of MSGs ( Supplementary Fig. S2 ). Table 2 Summary of the ChIP-PCR results. Full size table Perturbation network of key TFs Although the constructed regulatory module predicts interactions between TFs ( Fig. 1b ), the directions of regulation are not known. To find out these, the top 10 TFs and another two known memory-regulating TFs ( Id3 and Tbx21 , #12 and #19 in the list, Table 1 ) [6] , [15] , [25] were perturbed in CD8 + T cells in vitro by overexpression through retroviral transduction. 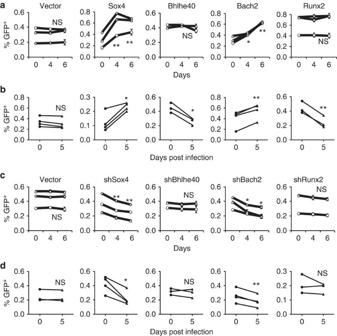Figure 3:Effect of overexpression and knockdown of TFs on memory CD8+T-cell recall proliferation. Naive 2C T cells were activatedin vitrowith SIY peptide and then transduced with retroviruses expressingSox4,Bhlhe40,Bach2orRunx2or expressing shRNA specific for one of the TFs. The cells were cultured in the presence of IL-7 to induce memory T-cell development. The resulting memory 2C T cells were either activatedin vitrowith SIY peptide or transferred into mice and activated by WSN-SIY virus infection. The proportion of GFP+(transduced) versus GFP−(non-transduced) 2C T cells was quantified 4 and 6 days post stimulationin vitroand in draining lymph node (DLN) 5 days post infection (dpi). Shown are proportions of GFP+2C T cells that overexpressedSox4,Bhlhe40,Bach2orRunx2among total 2C T cellsin vitro(a) andin vivo(b) or that expressed shRNA specific forSox4,Bhlhe40,Bach2orRunx2among total 2C T cells isin vitro(c) andin vivo(d). Each line was one independent experiment with one sample per time point for thein vitroexperiments and one or two mice perin vivoexperiment. Data shown are mean±s.e.m. Pairwise two-tailedt-tests were used for statistical analyses. *P<0.05; **P<0.01. NS, not significant. The transcript level of each of the 12-selected TFs was measured by quantitative real-time PCR ( Table 3 ). If changes in transcript level of more than twofold were taken as directional regulations, the perturbation results identified 41 regulations among the 12 × 12 matrix (31%). Notably, the top three TFs ( Sox4 , Tcf7 and Eomes ) directed 19 of the 41 regulations. To verify these regulations, ChIP-PCR was performed using antibodies specific for Sox4, Tcf7 and Eomes. As shown in Fig. 2a ( Supplementary Fig. S15 ), 18 of the 19 regulations were confirmed. ChIP-PCR also identified four more regulations that were not observed in the perturbation study. Thus, compared with ChIP-PCR, perturbation studies is able to identify the directional regulations with 82% sensitivity and 91% specificity. Table 3 Perturbation analysis. Full size table Figure 2: Construction of perturbation network of TFs in CD8 + T cells . ( a ) ChIP-PCR analysis. ChIP was carried out with 2C T cells using antibodies specific for Sox4, Tcf7 or Eomes or control IgG antibodies. Promoter regions of the indicted genes were then amplified using the precipitated DNA. Shown are PCR products after electrophoresis. ( b ) Perturbation network based on Table 3 . ( c ) An example of network motifs from the perturbation network. Full size image We then constructed a perturbation network of the 12 TFs with directional regulations ( Fig. 2b ). The top three TFs ( Sox4 , Tcf7 and Eomes ) and Bach2 had more downstream targets than the number of TFs that regulate them ( Supplementary Fig. S3 ), suggesting that they are at the upstream of a regulatory structure. TFs in the perturbation network formed multiple motifs, such as feedback and feed-forward loops ( Supplementary Fig. S4 ). For example, in a feedback motif of Sox4 - Tcf7 - Eomes - Tbx21 ( Fig. 2c ), Sox4 and Tcf7 regulate each other and they also regulate expression of Eomes and/or Tbx21 . The latter regulations were further confirmed at the protein level as indicated by suppression of Eomes and Tbx21 by overexpression of Sox4 or Tcf7 ( Supplementary Fig. S5 ). These results suggest that complex regulations involving multiple regulatory motifs among these TFs are involved in memory CD8 + T-cell development. Validation of Sox4 and Bach2 in memory CD8 + T cells Among the top 10 TFs ( Table 1 ), 6 are known to have important roles in memory CD8 + T-cell development and/or function. We then investigated whether the other four TFs ( Sox4 , Bhlhe40 , Bach2 and Runx2 ) are also involved in memory CD8 + T-cell development/function by examining the effect of overexpression and knockdown of these TFs on the recall proliferation of memory CD8 + T cells in vitro and in vivo . CD8 + T cells expressing the 2C TCR were activated with cognate peptide SIYRYYGL (SIY) and then transduced with retroviruses expressing GFP plus Sox4 , Bhlhe40 , Bach2 or Runx2 or expressing GFP plus shRNA specific for one of the four TFs ( Supplementary Tables S3 and S4 ). The 2C T cells were then cultured in the presence of cytokine IL-7 to induce the development of memory CD8 + T cells ( Supplementary Fig. S6 ). To assay recall proliferation, the in vitro memory 2C T cells were restimulated with SIY and the number of transduced (GFP + ) and non-transduced (GFP − ) 2C T cells were quantified on days 4 and 6. Compared with the vector control, overexpression of Sox4 or Bach2 led to a significant increase in the proportions of GFP + cells ( Fig. 3a ), suggesting a higher recall proliferation. When the in vitro generated memory 2C T cells were adoptively transferred into C57BL/6 (B6) mice followed by activation through infection with influenza virus that express SIY (WSN-SIY virus) [26] , a significant increase in the proportion of GFP + 2C T cells was also observed in the draining lymph nodes (DLN) ( Fig. 3b ), the blood, lung and spleen ( Supplementary Fig. S7 ) 5 days post infection (dpi) if the transduced memory T cells expressed Sox4 or Bach2 . Conversely, knockdown of Sox4 or Bach2 ( Supplementary Fig. S8 ) resulted in a significant inhibition of the recall proliferation of memory 2C T cells both in vitro and in vivo ( Fig. 3c,d ). Although overexpression of Bhlhe40 and Runx2 inhibited the in vivo recall proliferation of the transduced memory 2C T cells ( Fig. 3b ), no significant change was observed in in vitro recall response ( Fig. 3a ) and in knockdown assay ( Fig. 3c,d ). As positive controls, we tested in parallel known TFs: overexpression of Eomes promoted the recall proliferation whereas overexpression of Klf2 inhibited the recall proliferation ( Supplementary Fig. S9 ), consistent with previous reports [9] , [11] . These results show that Sox4 and Bach2 likely promote the recall proliferation of memory CD8 + T cells. Figure 3: Effect of overexpression and knockdown of TFs on memory CD8 + T-cell recall proliferation . Naive 2C T cells were activated in vitro with SIY peptide and then transduced with retroviruses expressing Sox4 , Bhlhe40 , Bach2 or Runx2 or expressing shRNA specific for one of the TFs. The cells were cultured in the presence of IL-7 to induce memory T-cell development. The resulting memory 2C T cells were either activated in vitro with SIY peptide or transferred into mice and activated by WSN-SIY virus infection. The proportion of GFP + (transduced) versus GFP − (non-transduced) 2C T cells was quantified 4 and 6 days post stimulation in vitro and in draining lymph node (DLN) 5 days post infection (dpi). Shown are proportions of GFP + 2C T cells that overexpressed Sox4 , Bhlhe40 , Bach2 or Runx2 among total 2C T cells in vitro ( a ) and in vivo ( b ) or that expressed shRNA specific for Sox4 , Bhlhe40 , Bach2 or Runx2 among total 2C T cells is in vitro ( c ) and in vivo ( d ). Each line was one independent experiment with one sample per time point for the in vitro experiments and one or two mice per in vivo experiment. Data shown are mean±s.e.m. Pairwise two-tailed t -tests were used for statistical analyses. * P <0.05; ** P <0.01. NS, not significant. Full size image Enhanced memory T-cell development by Bach2 overexpression To confirm the effect of overexpression of Bach2 on recall proliferation of memory CD8 + T cells, we activated 2C T cells in vitro for 2 days, transduced the activated T cells with retroviruses expressing GFP alone or GFP plus Bach2. The cells were cultured in the presence of IL-2 for 2 more days and then adoptively transferred into antigen-free B6 mice to induce in vivo memory 2C T cells ( Fig. 4a ). Twenty-three days after transfer, the frequency, phenotype and function of persisting 2C T cells were analysed. Both transduced (GFP + ) and non-transduced (GFP − ) 2C cells persisted in the recipient mice ( Fig. 4b ). GFP + 2C cells exhibited a typical memory phenotype as indicated by expression of CD62L and IL-7 receptor (IL-7R), similar to the GFP − 2C cells in the same recipient ( Fig. 4c ). The persisting memory 2C cells, both transduced and non-transduced, were rapidly induced to express IFNγ and TNFα following antigen stimulation ( Fig. 4d ). Furthermore, some recipient mice were infected with WSN-SIY virus and the recall proliferation of persisting 2C cells in the spleen and DLN were analysed 7 days later. As shown in Fig. 4e , if the 2C cells were originally transduced with GFP-expressing retrovirus, the proportion of GFP + versus GFP − 2C cells did not change following WSN-SIY challenge. However, if the 2C cells were originally transduced with GFP and Bach2 -expressing retrovirus, the proportion of GFP + cells was significantly higher in both DLN and spleen, suggesting a stronger recall proliferation by Bach2 -expressing memory 2C cells. 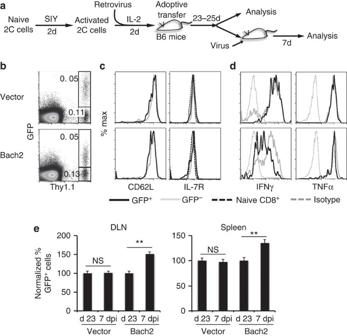Figure 4:Bach2promotes recall proliferation of memory CD8+T cells. (a) Scheme of experimental protocol. (b–d) Phenotype and function of persisting memory 2C cells. Twenty-two days post transfer, single-cell suspension was prepared from spleen and analysed for CD8, Thy1.1, GFP plus CD62L or IL-7R directly or stimulatedin vitrowith SIY peptide for 5 h before staining for CD8, Thy1.1, GFP plus intracellular IFNγ or TNFα. Comparison of GFP versus Thy1.1 (b) staining profiles of live cells between vector control andBach2overexpression group. Comparison of CD62L and IL-7R (c) or IFNγ and TNFα expression (d) between GFP+and GFP−2C T cells. Grey trace, non-transduced (GFP−) 2C T cells; black trace, transduced (GFP+) 2C T cells; dash grey trace, isotype control for intracellular staining; dash black trace, IL-7R staining of naive 2C T cells. (e) Recall responses of persisting memory 2C T cellsin vivo. Some recipient mice were infected with WSN-SIY 23–25 days post transfer and the proportions of GFP+and GFP−2C T cells in the DLN and spleen was quantified by flow cytometry 7 dpi. Comparison of proportions of GFP+2C T cells in the DLN and spleen before (d 23) and after antigen restimulation (7 dpi). Representative data from three independent experiments with 2–3 mice per group per experiment are shown as mean±s.e.m. Two-tailed Student’st-tests were used for statistical analyses. **P<0.01; NS, not significant. Figure 4: Bach2 promotes recall proliferation of memory CD8 + T cells . ( a ) Scheme of experimental protocol. ( b – d ) Phenotype and function of persisting memory 2C cells. Twenty-two days post transfer, single-cell suspension was prepared from spleen and analysed for CD8, Thy1.1, GFP plus CD62L or IL-7R directly or stimulated in vitro with SIY peptide for 5 h before staining for CD8, Thy1.1, GFP plus intracellular IFNγ or TNFα. Comparison of GFP versus Thy1.1 ( b ) staining profiles of live cells between vector control and Bach2 overexpression group. Comparison of CD62L and IL-7R ( c ) or IFNγ and TNFα expression ( d ) between GFP + and GFP − 2C T cells. Grey trace, non-transduced (GFP − ) 2C T cells; black trace, transduced (GFP + ) 2C T cells; dash grey trace, isotype control for intracellular staining; dash black trace, IL-7R staining of naive 2C T cells. ( e ) Recall responses of persisting memory 2C T cells in vivo . Some recipient mice were infected with WSN-SIY 23–25 days post transfer and the proportions of GFP + and GFP − 2C T cells in the DLN and spleen was quantified by flow cytometry 7 dpi. Comparison of proportions of GFP + 2C T cells in the DLN and spleen before (d 23) and after antigen restimulation (7 dpi). Representative data from three independent experiments with 2–3 mice per group per experiment are shown as mean±s.e.m. Two-tailed Student’s t -tests were used for statistical analyses. ** P <0.01; NS, not significant. Full size image The observed stronger recall response by Bach2 -expressing memory 2C cells could be due to the generation of more memory T cells and/or that the Bach2 -expressing memory T cells are more responsive to restimulation. To investigate these possibilities, we activated 2C T cells in vitro for 2 days and transduced them with retroviruses expressing GFP alone (vector) or GFP plus Bach2 ( Fig. 5a ). Twenty-four hours later, the T cells were adoptively transferred into B6 mice followed by WSN-SIY virus infection. 2C T-cell responses were analysed by flow cytometry 7 dpi. Compared with the non-transduced 2C T cells, vector-transduced 2C T cells had the same expression profiles for CD62L, IL-7R, Klrg1 and CD27 in the same organs of the same mice ( Fig. 5b , upper panel). In contrast, a significantly higher proportion of Bach2 -transduced 2C T cells expressed CD62L and CD27, but a significantly lower fraction expressed Klrg1, in the DLN and spleen compared with non-transduced 2C cells in the same organs of the same recipients. When the persisting 2C T cells were analysed on 30 dpi, no significant differences in IFNγ and IL-2 expression were observed among non-transduced, vector-transduced and Bach2 -transduced 2C T cells in response to restimulation in vitro ( Fig. 5c and Supplementary Fig. S10 ). Although no difference in CD62L and IL-7R expression was detected, CD27 was higher in Bach2 -transduced than vector-transduced 2C T cells in the lung and DLN. ( Fig. 5c and Supplementary Fig. S10 ). Importantly, significantly more Bach2 -transduced 2C T cells persisted in the DLN, spleen and bone marrow ( Fig. 5d,e ). These result suggest that overexpression of Bach2 likely promotes the generation of memory CD8 + T cells in vivo . 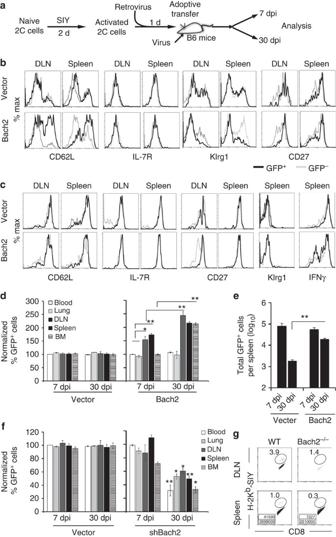Figure 5:Bach2promotes memory CD8+T-cell development. (a) Scheme of experimental protocol forb–f. (b–e) Effect of Bach2 overexpression on memory T-cell development. (b,c) Persistence and phenotype of transferred 2C T cells over time. Seven and 30 dpi, 2C T cells in various organs were analysed for CD62L, IL-7R, Klrg1, CD27 and IFNγ as inFig. 4. Shown are histograms of CD62L, IL-7R, Klrg1 and CD27 expression of Thy1.1+CD8+2C T cells 7 (b) and 30 dpi (c). Grey trace, non-transduced (GFP−) 2C T cells; black trace, transduced (GFP+) 2C T cells. Representative data from six mice in three independent experiments are shown. (d) Proportion of GFP+transduced 2C cells in different organs normalized to the average of the blood at 7 dpi. (e) Total Bach2-transduced 2C T cells (GFP+) in the spleen 7 and 30 dpi. (f) Effect of Bach2 knockdown on memory T-cell development. Proportion of Bach2-knocked down 2C T cells (GFP+) in different organs normalized to the average of the blood at 7 dpi. (g) Effect of Bach2 knockout on memory T-cell development. Chimera mice were constructed by injecting Bach2−/−and Bach2+/+bone marrow cells into sublethally irradieated Rag2−/−recipient mice. Following reconstitution (3 months later), mice were infected with WSN-SIY virus and 30 dpi cells from DLN and spleen were stained for H-2Kb-SIY and anti-CD8. Shown are staining profiles of H-2Kb-SIY versus CD8. The numbers in the plots indicate percentage of SIY-specific memory CD8+T cells. The numbers in the boxes indicate the number of SIY-specific memory CD8+T cells (top) and total CD8+T cells (bottom). Representative data from three independent experiments with 2–3 mice per group per experiment (d,e) and from two independent experiments with 3–4 mice per group per experiment (f) are shown as mean±s.e.m. Two-tailed Student’st-tests were used for statistical analyses. *P<0.05; **P<0.01. Figure 5: Bach2 promotes memory CD8 + T-cell development . ( a ) Scheme of experimental protocol for b – f . ( b – e ) Effect of Bach2 overexpression on memory T-cell development. ( b , c ) Persistence and phenotype of transferred 2C T cells over time. Seven and 30 dpi, 2C T cells in various organs were analysed for CD62L, IL-7R, Klrg1, CD27 and IFNγ as in Fig. 4 . Shown are histograms of CD62L, IL-7R, Klrg1 and CD27 expression of Thy1.1 + CD8 + 2C T cells 7 ( b ) and 30 dpi ( c ). Grey trace, non-transduced (GFP − ) 2C T cells; black trace, transduced (GFP + ) 2C T cells. Representative data from six mice in three independent experiments are shown. ( d ) Proportion of GFP + transduced 2C cells in different organs normalized to the average of the blood at 7 dpi. ( e ) Total Bach2-transduced 2C T cells (GFP + ) in the spleen 7 and 30 dpi. ( f ) Effect of Bach2 knockdown on memory T-cell development. Proportion of Bach2-knocked down 2C T cells (GFP + ) in different organs normalized to the average of the blood at 7 dpi. ( g ) Effect of Bach2 knockout on memory T-cell development. Chimera mice were constructed by injecting Bach2 −/− and Bach2 +/+ bone marrow cells into sublethally irradieated Rag2 −/− recipient mice. Following reconstitution (3 months later), mice were infected with WSN-SIY virus and 30 dpi cells from DLN and spleen were stained for H-2K b -SIY and anti-CD8. Shown are staining profiles of H-2K b -SIY versus CD8. The numbers in the plots indicate percentage of SIY-specific memory CD8 + T cells. The numbers in the boxes indicate the number of SIY-specific memory CD8 + T cells (top) and total CD8 + T cells (bottom). Representative data from three independent experiments with 2–3 mice per group per experiment ( d , e ) and from two independent experiments with 3–4 mice per group per experiment ( f ) are shown as mean±s.e.m. Two-tailed Student’s t -tests were used for statistical analyses. * P <0.05; ** P <0.01. Full size image We further investigated the effect of Bach2 overexpression in naive 2C T cells on memory CD8 + T-cell development in vivo . Bone marrow progenitor cells isolated from 2C TCR transgenic mice were transduced with retroviruses expressing GFP alone or GFP plus Bach2 and adoptively transferred into sublethally irradiated Rag2 −/− mice to generate naive 2C T cells that express GFP or GFP plus Bach2 ( Fig. 6a ). The resulting transduced and non-transduced naïve 2C cells were then adoptively transferred into B6 mice followed by infection with WSN-SIY virus. The frequency, phenotype and function of 2C T cells were analysed on 7 dpi. Vector-transduced and non-transduced 2C T cells from the same recipient mice had the same expression profile of CD62L, IL-7R, Klrg1, IFNγ and TNFα ( Fig. 6b ). While Bach2 -transduced 2C T cells expressed similar levels of IFNγ and TNFα as non-transduced and vector-transduced 2C T cells, more cells expressed CD62L but fewer cells expressed Klrg1, resembling to CD62L hi Klrg1 low memory precursors ( Fig. 6b and Supplementary Fig. S11 ). By 30 dpi, no significant differences were observed among non-transduced, vector-transduced and Bach2 -transduced 2C T cells in expression of CD62L, IL-7R, Klrg1, IFNγ and TNFα ( Fig. 6c ). However, more Bach2 -transduced 2C T cells were found in the blood, lung, DLN and spleen 30 dpi ( Fig. 6d,e ). Together, these data suggest that overexpression of Bach2 promotes the development of memory CD8 + T cells. 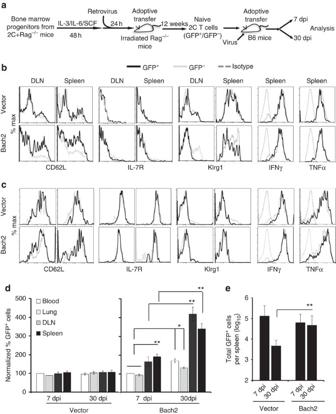Figure 6:Bach2promotes memory CD8+T-cell development. (a) Scheme of experimental protocol. (b–e) Persistence and phenotype of transferred CD8+T cells over time. Seven and 30 dpi, 2C T cells in various organs were analysed as inFig. 4. Shown are histograms of CD62L, IL-7R, Klrg1, IFNγ and TNFα expression of Thy1.1+CD8+2C T cells 7 (b) and 30 dpi (c). Grey trace, non-transduced (GFP−) 2C T cells; black trace, transduced (GFP+) 2C T cells; dash grey trace, isotype control for intracellular staining. Representative data from 9–12 mice in three independent experiments are shown. (d) Proportion of GFP+transduced 2C cells in different organs normalized to the average of the blood at 7 dpi. (e) Total Bach2-transduced 2C T cells (GFP+) in the spleen 7 and 30 dpi. Data from three independent experiments with 3–4 mice per group per experiment are shown as mean±s.e.m. Two-tailed Student’st-tests were used for statistical analyses. *P<0.05; **P<0.01. Figure 6: Bach2 promotes memory CD8 + T-cell development . ( a ) Scheme of experimental protocol. ( b – e ) Persistence and phenotype of transferred CD8 + T cells over time. Seven and 30 dpi, 2C T cells in various organs were analysed as in Fig. 4 . Shown are histograms of CD62L, IL-7R, Klrg1, IFNγ and TNFα expression of Thy1.1 + CD8 + 2C T cells 7 ( b ) and 30 dpi ( c ). Grey trace, non-transduced (GFP − ) 2C T cells; black trace, transduced (GFP + ) 2C T cells; dash grey trace, isotype control for intracellular staining. Representative data from 9–12 mice in three independent experiments are shown. ( d ) Proportion of GFP + transduced 2C cells in different organs normalized to the average of the blood at 7 dpi. ( e ) Total Bach2-transduced 2C T cells (GFP + ) in the spleen 7 and 30 dpi. Data from three independent experiments with 3–4 mice per group per experiment are shown as mean±s.e.m. Two-tailed Student’s t -tests were used for statistical analyses. * P <0.05; ** P <0.01. Full size image Diminished memory T-cell development due to Bach2 deficiency We also examined the effect of Bach2 knockdown on memory T-cell development. The approach was the same as outlined as in Fig. 5a , except the retrovirus expressed shRNA specific for Bach2. Briefly, activated 2C T cells were transduced with shRNA-expressing retrovirus and adoptively transferred into B6 mice followed by infection with WSN-SIY influenza virus. The number and frequency of GFP + and GFP − 2C T cells in various organs were analysed on 7 and 30 dpi. No significant difference was observed among non-transduced, vector-transduced and shRNA-transduced 2C T cells in terms of CD62L, IL-7R, Klrg1, CD27 and IFNγ expression ( Supplementary Fig. S12 ). However, the proportion of shRNA-transduced 2C T cells was reduced significantly in the blood, lung, DLN, spleen and bone marrow 30 but not 7 dpi ( Fig. 5f ). Consistently, the number of shRNA-transduced 2C T cells in the spleen was lower as compared with the numbers of non-transduced and vector-transduced 2C T cells 30 dpi ( Supplementary Fig. S12c ). To investigate the effect of Bach2 knockout on memory T-cell development, we constructed chimeric mice where T and B cells were deficient in Bach2 by adoptively transferring bone marrow cells from Bach2 knockout mice into sublethally irradiated Rag2 −/− mice. Three months after reconstitution, mice were infected with WSN-SIY influenza virus and analysed for the presence of SIY-specific memory CD8 + T cells 30 days later. The percentage of SIY-specific CD8 + T cells was lower in the DLN and spleen of chimeric mice that were reconstituted with Bach2 −/− than Bach2 +/+ bone marrow cells ( Fig. 5g ). Consistently, the number of SIY-specific CD8 + T cells in the spleen was lower in mice reconstituted with Bach2 −/− than Bach2 +/+ bone marrow cells. Considering that Bach2 expression was downregulated in effector and then upregulated in memory T cells during naive to effector to memory cell transition ( Table 1 ), together these results show that Bach2 promotes memory CD8 + T-cell development. Enhanced proliferation of T cells by Bach2 overexpression To further explore the mechanism underlying the observed effect of Bach2 on memory T-cell development and response, we examined whether Bach2 affects T-cell proliferation. 2C T cells were activated in vitro and transduced with either vector or Bach2 -expressing retroviruses. The cells were cultured in the presence of either IL-2 or IL-7 and the proportion of transduced (GFP + ) versus non-transduced (GFP − ) cells in the same cultures was quantified over time. In the IL-7 culture, the proportion of transduced versus non-transduced 2C cells remained stable regardless of whether the 2C T cells were transduced with vector or Bach2 ( Fig. 7a ). Similarly, the proportion of vector-transduced versus non-transduced 2C cells remained stable in the IL-2 cultures. However, the proportion of Bach2 -transduced 2C T cells increased significantly over time in the IL-2 cultures ( Fig. 7a ). When the cells were lableled with eFluor and followed over time, Bach2 -transduced 2C T cells diluted the flourescent dye more extensively than non-transduced 2C T cells ( Fig. 7b ). These data suggest that Bach2 promotes proliferation of activated CD8 + T cells. 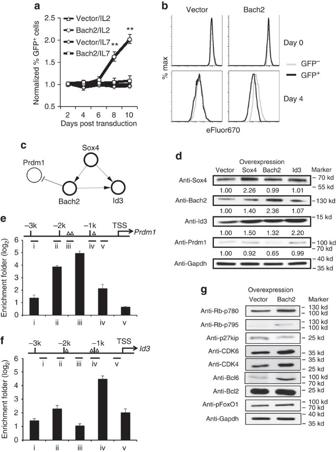Figure 7:Bach2promotes proliferation of CD8+T cells. (a) 2C cells were activatedin vitroand transduced with retroviruses expressing GFP alone (vector) or GFP plus Bach2 and cultured in the presence of either IL-2 or IL-7. The proportion of GFP+2C T cells was quantified. Shown (mean±s.e.m.) are changes in proportion of GFP+cells over time from four independent experiments. Two-tailed student’st-tests were used for statistical analyses. **P<0.01. (b)Bach2-transduced 2C T cells (day 4 ina) were labelled with eFluor670 and cultured in the presence of IL-2 for 4 days. Shown are representative histograms of eFluor670 from one of the two experiments. Grey trace, non-transduced (GFP−) 2C T cells; black trace, transduced (GFP+) 2C T cells. (c)Sox4-Bach2-Prdm1-Id3regulatory motif identified in perturbation network. (d) Bach2 inhibits Prdm1 expression but promotes Id3 expression. Activated 2C T cells were transduced with retroviruses expressing GFP alone (vector) or GFP plusBach2,Sox4orId3. The levels of the indicated TFs were assayed by western blotting. Shown are representative western blotting and the average expression level quantified from three independent experiments. (e,f) Bach2 binds toPrdm1andId3promoter. Activated 2C T cells were cultured with IL-7 for 24 h and harvested for ChIP using anti-Bach2. DNA was used to amplify different parts of thePrdm1(e) andId3(f) promoter region indicated by (i–v). The location of the predicted Bach2 binding motif was indicted as triangle. Data are from two independent experiments, error bar: s.e.m. (g)Bach2affects Rb phosphorylation and p27kip expression. Activated 2C T cells were transduced with retroviruses expressing GFP alone (vector) or GFP plus Bach2 and cultured for 8 days (a). The levels of phosphorylated Rb and FoxO1, CDK4, CDK6, Bcl6, Bcl2 and p27kip in the transduced 2C T cells were assayed by western blotting. Figure 7: Bach2 promotes proliferation of CD8 + T cells . ( a ) 2C cells were activated in vitro and transduced with retroviruses expressing GFP alone (vector) or GFP plus Bach2 and cultured in the presence of either IL-2 or IL-7. The proportion of GFP + 2C T cells was quantified. Shown (mean±s.e.m.) are changes in proportion of GFP + cells over time from four independent experiments. Two-tailed student’s t -tests were used for statistical analyses. ** P <0.01. ( b ) Bach2 -transduced 2C T cells (day 4 in a ) were labelled with eFluor670 and cultured in the presence of IL-2 for 4 days. Shown are representative histograms of eFluor670 from one of the two experiments. Grey trace, non-transduced (GFP − ) 2C T cells; black trace, transduced (GFP + ) 2C T cells. ( c ) Sox4-Bach2-Prdm1-Id3 regulatory motif identified in perturbation network. ( d ) Bach2 inhibits Prdm1 expression but promotes Id3 expression. Activated 2C T cells were transduced with retroviruses expressing GFP alone (vector) or GFP plus Bach2 , Sox4 or Id3 . The levels of the indicated TFs were assayed by western blotting. Shown are representative western blotting and the average expression level quantified from three independent experiments. ( e , f ) Bach2 binds to Prdm1 and Id3 promoter. Activated 2C T cells were cultured with IL-7 for 24 h and harvested for ChIP using anti-Bach2. DNA was used to amplify different parts of the Prdm1 ( e ) and Id3 ( f ) promoter region indicated by (i–v). The location of the predicted Bach2 binding motif was indicted as triangle. Data are from two independent experiments, error bar: s.e.m. ( g ) Bach2 affects Rb phosphorylation and p27kip expression. Activated 2C T cells were transduced with retroviruses expressing GFP alone (vector) or GFP plus Bach2 and cultured for 8 days ( a ). The levels of phosphorylated Rb and FoxO1, CDK4, CDK6, Bcl6, Bcl2 and p27kip in the transduced 2C T cells were assayed by western blotting. Full size image We noticed a feed-forward regulatory motif of Sox4-Bach2-Prdm1-Id3 in the perturbation network ( Fig. 7c and Supplementary Fig. S4 ). We verified this regulatory motif by showing that overexpression of Bach2 suppressed expression of Prdm1 but stimulated expression of Id3 at transcriptional ( Table 3 ) and translational levels ( Fig. 7d ; Supplementary Fig. S16 ). ChIP-PCR analysis with anti-Bach2 antibody also confirmed that Bach2 binds directly to the promoter regions of Prdm1 and Id3 ( Fig. 7e,f ). Further supporting the regulatory motif, overexpression of Prdm1 significantly reduced the Bach2 -mediated proliferation of activated T cells ( Supplementary Fig. S13 ). As Prdm1 is known to inhibit T-cell proliferation whereas Id3 stimulates survival of effector T cells [15] , [16] , we determined the effect of Bach2 overexpression on molecules that regulate cell cycle and survival. Overexpression of Bach2 stimulated CDK4, CDK6 and Bcl6 expression and Rb phosphorylation at amino acid residues 780 and 795 but inhibited expression of p27kip ( Fig. 7g ; Supplementary Fig. S16 ). These results suggest that Bach2 regulates memory T-cell development and recall proliferation by regulating cell cycle control possibly through Prdm1 and Id3 . At the molecular level, development of memory CD8 + T cells is the establishment of MSG expression programme, which ultimately is controlled by TFs. Although several TFs have been described to regulate memory CD8 + T-cell development, for a comprehensive understanding of transcriptional regulation of memory CD8 + T-cell development, it is necessary to identify most, if not all, key TFs that regulate MSGs and construct a genome-wide transcriptional network that supports memory CD8 + T-cell development. Using systems biology approaches and publically available gene expression data, here we have assembled a genome-wide regulatory network associated with CD8 + T cells of the mouse. Applying MRA to this network, we have identified 21 key TFs, down-narrowed from 1,038 putative TFs, which regulate the expression of 70% of MSGs. Our approach is valid based on the following considerations. First, our method identified 8 of the 12 TFs known to be involved in memory CD8 + T-cell development, including Tcf7 , Eomes , Prdm1 , Klf2 , Id2 , Stat4 , Id3 and Tbx21 ( Table 1 ). Although Bcl6 , Stat3 and Myc are known to regulate memory CD8 + T-cell development, they were not within the top 21 TFs identified using our methodology because CLR-inferred targets do not overlap with MSGs possibly due to limited data on MSGs or the network. NF-κb has important roles in both effector and memory T-cell development [27] , [28] . We found that NF-κb was a key TF that regulates effector signature genes when MRA was applied to the network and effector signature genes. Second, our method identified several TFs that are not known to function in the memory CD8 + T-cell development, including Sox4 , Bhlhe40 , Bach2 and Runx2 in the top 10 TFs ( Table 1 ). Follow-up experimentation showed that these newly identified TFs indeed have important roles in memory CD8 + T-cell development and function. Overexpression of Sox4 and Bach2 promoted a significantly higher recall proliferation of memory CD8 + T cells both in vitro and in vivo . Conversely, knockdown of Sox4 and Bach2 inhibited the recall proliferation of the transduced memory T cells ( Fig. 3 ). Overexpression of Bhlhe40 and Runx2 inhibited the in vivo recall proliferation, although no significant change was observed in in vitro recall response and in knockdown assay ( Fig. 3 ). Further analysis showed that overexpression of Bach2 also promotes memory CD8 + T-cell development ( Figs 4 , 5 , 6 ). Third, compared with the traditional method of differential gene expression analysis [2] , [3] , which generates a long list of candidates using fold-change-based approaches, our network methods identify and rank order TFs according to their statistical importance. Reduction of hundreds of TFs to two-dozen key TFs makes direct experimental validation more manageable. The network approach and methodologies developed here can be applied to any phenotypic transition, such as effector T cells and exhausted T cells, to identify novel transcriptional modules and TFs. Studies have suggested that memory CD8 + T-cell development is coordinately regulated by several TFs (reviewed in refs 22 , 24 ), including Eomes and Tbx21 (ref. 4 ). Our network and perturbation studies have now greatly expanded the understanding of the mode of interactions to the top 21 TFs. Our analysis reveals a dense overlapping regulation among the key TFs ( Fig. 2b ). This mode of regulation is essential for sensing multiple external signals and integrate them into distinct cell fate outcomes [29] . As two classes of TFs have been proposed to control the developmental potentials of effector and memory fates in a quantitative manner [22] , [24] , [30] , the dense overlapping regulation might contribute to the quantitative regulations during effector to memory CD8 + T-cell development. Our analysis also shows complex regulations with both feedback and feed-forward motifs among the key TFs ( Table 3 and Fig. 2b ). In the regulatory motif of Sox4 - Tcf7 - Eomes - Tbx21 , Tcf7, Eomes and Tbx21 are known to be critical for memory CD8 + T-cell development. The association of Sox4 with these three TFs and especially its ‘hub’ position in this motif are intriguing. Sox4 is not known to regulate memory CD8 + T-cell development. However, it stabilizes β-catenin to modulate Wnt-Tcf7 signalling [31] , [32] , which promotes memory CD8 + T-cell development. Sox4 also regulates ‘stemness’ of cancer cells [33] , a property shared by memory T cells. Furthermore, evidence suggests that Sox4 might be a direct regulatory target of TGFβ signalling [34] , which is essential for the differentiation of CD8 + T cells [35] . These previous observations, together with our finding of the ‘hub’ position of Sox4 in the regulatory motif of Sox4 - Tcf7 - Eomes - Tbx21 , suggest that Sox4 is a critical TFs regulating memory CD8 + T-cell development. While this hypothesis has yet to be validated, our finding that overexpression of Sox4 promotes recall proliferation of memory T cells suggests that Sox4 is involved in memory CD8 + T-cell development. In the regulatory motif of Sox4 - Tcf7 - Eomes - Tbx21 , we found that Tcf7 binds to Eomes promoter ( Fig. 2a ) and retroviral expression of Tcf7 leads to a downregulation of Eomes transcript ( Table 3 ) and protein ( Supplementary Fig. S5 ). The latter results contradict with the previous report showing that the level of Eomes transcript and protein are decreased in memory CD8 + T cells from Tcf7-deficient mice [9] . Although we do not know the precise causes underlying the observed opposite effects, the following differences between the two studies may provide part of the explanation. First, our study was carried out in in vitro , using activated CD8 + T cells that are in transition to memory T cells, whereas the previous study used memory CD8 + T cells directly from mice. Second, in our study, we overexpressed Tcf7 for a short period (72 h) before assaying the effect on Eomes expression, whereas the previous study examined the accumulated effect of germline Tcf7 knockout on Eomes expression. The differences in the stage of T cells, in vitro versus in vivo , overexpression versus deficiency, and the length of Tcf7 overexpression or deficiency could all contribute to the observed differences in the two studies. Although the discrepancy raises concern of our approach, results from our perturbation study on the effect of Bach2 on Prdm1 , Prdm1 on Tcf7 and Id2 on Id3 are all consistent with previous reports [17] , [36] , [37] , suggesting the validity of our in vitro assay in most cases. Our detailed analysis of the feed-forward motif of Sox4-Bach2-Prdm1-Id3 ( Fig. 7c ) reveals new insight into memory CD8 + T-cell development. This regulatory motif includes two known TFs ( Id3 and Prdm1 ) and two unknown TFs ( Sox4 and Bach2 ) in memory CD8 + T-cell development. Through both overexpression and knockdown/knockout in CD8 + T cells both in vitro and in mice, we provide extensive evidence showing that Bach2 promotes memory CD8 + T-cell development ( Figs 4 , 5 , 6 ). One mechanism appears to be stimulating the induction of memory T-cell precursors as Bach2 expression in effector T cells leads to a phenotype of CD62L hi Klrg lo CD27 + ( Fig. 5b,c and Supplementary Fig. S10 ), which are considered as central memory T-cell precursors with high proliferative potential [38] , [39] . Recently, two studies report that Bach2 regulates CD4 + T-cell development and function by suppressing effector gene expression [40] , [41] . Our observation that Klrg1 is suppressed by Bach2 suggests that suppression of effector function may also be important for the development of memory CD8 + T cells. Another mechanism is by stimulating T-cell proliferation. We showed that overexpression of Bach2 enhances IL-2 driven T-cell proliferation in vitro and recall proliferation in vitro and in vivo . In addition, when in vitro memory 2C T cells were labelled with eFluro dye and adoptively transferred into Rag −/− mice, Bach2 -transduced T cells diluted the flourescent dye more extensively than the non-transduced and vector-transduced T cells ( Supplementary Fig. S14 ). The enhanced proliferation could lead to development and/or survival of memory T cells. Our study further sheds light on the mechanisms by which Bach2 promotes T-cell proliferation. In the regulatory motif, Bach2 promotes Id3 expression but suppresses Prdm1 expression through direct binding to their promoter regions ( Fig. 7c–f ); the latter is consistent with Bach2 suppression of Prdm1 expression in B cells [37] . Id3 is known to promote cell cycle and recall proliferation of memory CD8 + T cells by binding to and inhibiting E proteins [15] , [42] . Thus, by promoting Id3 expression, Bach2 stimulates T-cell proliferation. Prdm1 is known to antagonize Bcl6 , which promotes cell cycle by suppressing the expression of cell cycle inhibitor p27kip [43] . Bcl6 −/− mice exhibit a profound deficiency of memory T cells [44] , [45] , whereas in the absence of p27kip, memory CD8 + T cells exhibit enhanced homoeostatic and recall proliferation [46] . Consistently, we show that overexpression of Bach2 promotes Bcl6 expression but inhibits p27kip expression ( Fig. 7g ). Thus, Bach2 also stimulates T-cell proliferation by suppressing Prdm1 expression. Together, these findings suggest that Bach2 promotes memory CD8 + T-cell development and recall proliferation through Id3- and Prdm1-mediated cell cycle control. Development of memory CD8 + T cells requires integration of multiple external and internal signals to establish a new transcriptional programme of MSGs that endows memory CD8 + T cells with characteristic features in phenotype, tissue distribution, homoeostasis and recall potentials. In this study, we have shown that integrated systems biology approaches can be effectively used to identify key TFs and their mode of interactions that underlies memory CD8 + T-cell differentiation and function. Further analysis of motifs in the regulatory network should help to elucidate in detail the molecular mechanisms underlying memory CD8 + T-cell development and function. Regulatory network and MRA A total of 386 public microarrays related to CD8 + T cells from 35 independent GEO data sets (till September 2009) were downloaded from the NCBI database of Gene Expression Omnibus (GEO) ( Supplementary Table S1 ). All raw image files were reprocessed to normalize the data using R programme with a gcRMA method. Gene expression data was used to construct the regulatory network with the putative TFs using a reverse-engineering algorithm CLR [19] . Among the 1,445 putative TFs identified according to the domain predictions of protein sequences [18] , 1,038 were manually mapped to the latest mouse genome. To compare gene expression in different CD8 + T cells, samples were grouped into naive, effector and memory based on the cell types from which the microarray analysis were done ( Supplementary Table S1 ). Gene was considered to be expressed in CD8 + T cells if the average gene expression level in one of the three groups was >8 (gcRMA values). To identify TFs associated with memory CD8 + T-cell development, we used MRA to compute the statistical significance of overlaps of all interactions of each TF (inferred by CLR) with MSGs or a control gene set by a binomial test. The MSGs were differentially expressed genes between memory CD8 + T cells and naive/effector CD8 + T cells identified previously [3] . 332 background genes were identified from the 386 gene expression profiles based on high levels of gene expression (gcRMA value >10) but minimal variation among 386 samples (variation from mean <0.5). This criterion minimizes the potential of the selected genes not being regulated by TFs in CD8 + T cells. From the 1,038 putative TFs, MRA identified 60 MSG-specific TFs at P <0.05 (binomial test), all of which are expressed in CD8 + T cells ( Supplementary Table S2 ). These 60 candidates were filtered by removing those whose knockout does not have any immune system phenotype as defined in MGI [20] . The positive candidates were analysed for enrichment of DNA-binding motifs in the promoter regions (−2,000 to −1) of the MSGs using the programme MatInspector [47] or differential expression among naive, effector and memory CD8 + T cells. This led to 21 key TFs that exhibit immune system phenotype with either an enrichment of DNA-binding motifs among MSGs or differential expression. Mice and virus The 2C TCR transgenic mice on Rag2 −/− and C57BL/6 (B6 Thy1.1 + ) background (2C + Rag −/− ) were maintained in the animal facility at the Massachusetts Institute of Technology (MIT). These mice express the 2C TCR on CD8 + T cells specific for SIYRYYGL peptide (SIY) in association with MHC class I K b molecule [48] . B6 and Rag2 −/− mice were from the Jackson Laboratory. Mice were used at 8–16 weeks of age. All animal studies and procedures were approved by the Massachusetts Institute of Technology’s Committee for Animal Care. Recombinant WSN-SIY virus encoding the SIY epitope in the neuroaminidase stalk was constructed by plasmid-based reverse genetics and grown in Madin–Darby canine kidney cells [26] . For infection, mice were anesthetized and given 100 p.f.u. (sublethal dose) intranasally. Flow cytometry and cell sorting Antibodies specific for CD8α, Thy1.1, Klrg1, CD62L, CD127 (IL-7R), CD27, IFNγ, TNFα, IL-2, Eomes and T-bet (Tbx21) were purchased from BioLegend or eBiosciences and used at the recommended concentration. Single-cell suspensions were prepared from spleens and mediastinal (draining) lymph nodes (DLN), peripheral blood and lung. Splenocytes and lymphocytes were collected in 8 ml HBSS by crushing the spleen and lymph node with frosted glass slides and filtering the cell suspension through 80-μm nylon filters, respectively. Lungs were collected and ground through a cell strainer, followed by incubation with 2 ml of digestion buffer (RPMI 1640 medium containing 3 mg ml −1 of collagenase A (Roche), 5% FBS and 10 mM HEPES) at 37 °C for 1 h. Red blood cells in the spleen, blood and lung were lysed with red blood cell lysis buffer (Gibco) and the cells were washed with complete RPMI. The cells were counted and 1–3 × 10 6 cells were used for surface staining. Cells were washed twice with PBS plus 2% FBS before cytometry analsysis. For intracellular staining, splenocytes were stimulated with SIY peptide for 5 h in the presence of GolgiPlug (BD Biosciences). Cells were washed twice with PBS with 2% FBS and stained with indicated antibodies. The cells were then fixed and stained with labelled antibodies using an intracellular staining kit (Cytofix/Cytoperm kit; BD Biosciences) according to the manufacturer’s instructions. Stained cells were analysed on either a FACSCalibur or Accuri C6 flow cytometer (BD Biosciences). About 0.5–2 × 10 6 events were collected and analysed with FlowJo software. Cell sorting was carried out with a MoFlo cell sorter or FACSAria (BD Biosciences). Retrovirus production and infection Retroviral pMIGw-GW gateway vector was constructed by inserting a gateway cassette at EcoRI site of the pMIGw vector (Addgene #9044) using a gateway construction kit (Invitrogen). All ORFs encoding 12 TFs were amplified with primers ( Supplementary Table S3 ) and cDNA from mouse splenocytes and cloned into pMIGw-GW using the gateway cloning technology. shRNAs for specific TFs ( Supplementary Table S4 ) were chosen from the predicted TRC library and cloned into pMKO.1 GFP retroviral vector (Addgene #10676). Briefly, synthesized single-strand sense and antisense oligonucleotides were annealed into double-strand oligonucleotides for short hairpin RNA in the annealing buffer (10 mM TrisCl (pH7.5), 50 mM NaCl and 1 mM EDTA). The double-strand oligonucleotides were directly treated with T4 polynucleotide kinase (NEB) and ligated into pMKO.1 GFP vector) between Age I and Eco RI sites. 293FT cells were cultured to 60% confluency in six-well plates. Cells were co-transfected with retroviral vector plasmid (4 μg) and packing plasmids pCL-Eco (1 μg) with 150 μl DMEM and 15 μl TransIT-LT1 (Mirus) according to the manufacturer’s instructions. On the second day, the culture was replaced with fresh medium. On the third day, supernatant was collected and filtered through a 0.45-μm low-protein binding membrane (Pall Life Science). Fresh viral supernatants were used for spin infection of CD8 + T cells in all experiments. For infection, cells from spleens and lymph nodes were harvested from 2C + RAG −/− mice, pooled and cultured in six-well plates in the presence of SIY peptide (1 μg ml −1 ) in the complete RPMI medium (RPMI 1640 supplemented with 10% FBS, 5 mM HEPES, 2 mM glutamine, 100 U ml −1 penicillin, 100 μg ml −1 streptomycin and 50 μM β-mercaptoethanol (Invitrogen)). Two days later, activated 2C T cells were collected, washed and resuspended at 2 × 10 6 cells per ml in the complete RPMI medium. Fresh retrovirus supernatants (1 ml) and 0.25 ml 2C cells with a final concentration of 5 μg ml −1 polybrene (American Bioanalytical) were added to one well of a 24-well plate and spun for 90 min at 2500, r.p.m. at 32 °C to infect T cells. Twenty four hours later, cells were collected for direct adoptive transfer, or resuspended and cultured in 3 ml fresh RPMI medium with 100 U ml −1 IL-2 (eBioscience). After being cultured for 24 h, 2C T cells were analysed for GFP expression by flow cytometry and prepared for injection into mice to generate in vivo memory T cells or further cultured to generate in vitro memory T cells. Generation and recall proliferation of memory T cells To generate in vitro memory T cells, activated (and transduced) 2C T cells were cultured in complete RPMI medium supplemented with 5 ng ml −1 IL-7 (Peprotech) for 7 days with change of fresh IL-7-supplemented medium every 2 days. Cells were analysed for memory phenotype by flow cytometry on day 7. To test the recall proliferation, in vitro memory 2C T cells (1 × 10 5 ) were cultured with B6 splenocytes (5 × 10 5 ) in a 12-well plate in complete RPMI medium supplemented with 1 μg ml −1 SIY peptide and 100 units per ml IL-2. The numbers and phenotype of 2C T cells were analysed by flow cytometry 4 and 6 days later. Alternatively, in vitro memory 2C T cells (2 × 10 5 ) were transferred to B6 recipients and challenged with WSN-SIY virus. 2C cells were analysed by flow cytometry 5 dpi. To generate in vivo memory T cells, activated and transduced 2C T cells were adoptively transferred into B6 recipients. Twentythree days later, the frequency, phenotype and function of persisting 2C T cells were analysed by flow cytometry. To assay for recall response, mice were infected with 100 p.f.u. WSN-SIY virus and the number and phenotype of 2C T cells in different organs were analysed by flow cytometry 7 dpi. Bone marrow chimera mice Bone marrow cells were collected from the tibia and femur of 2C + Rag −/− mice. Stem and progenitor cells were enriched using a progenitor enrichment kit (Stemcell Technologies) according to the manufacturer’s instructions. The enriched cells were cultured for 48 h in complete RPMI medium supplemented with IL-3 (30 ng ml −1 ), IL-6 (10 ng ml −1 ) and SCF (15 ng ml −1 ). The cells were resuspended at 2 × 10 6 cells per ml in complete RPMI. Fresh retrovirus supernatants (600 μl) and 400 μl cells plus a final concentration of 6 μg ml −1 polybrene were added to one well of a 24-well plate and spun for 90 min at 2,500 r.p.m. at 32 °C. One the second day, cells were collected and washed and injected into Rag −/− mice that had been irradiated for 500 rads 4 h earlier. Eight weeks later, mice were bleeded to determine the reconstitution of CD8 + T cells and GFP proportion by flow cytometry. Twelve weeks later, cells were collected from spleen and analysed for 2C T-cell percentage and phenotype. Splenocytes containing 5 × 10 4 2C T cells were adoptively transferred into B6 mice followed by WSN-SIY infection. The number, phenotype and function of 2C T cells in the recipient mice were analysed on 7 and 30 dpi. To generate Bach2 −/− chimeric mice, bone marrow cells from Bach2 −/− mice [49] (kind gift of Dr Kazuhiko Igarash of Tohoko University, Japan) were directly injected into sublethally irradiated Rag2 −/− mice. Eight weeks later, reconstitution of CD8 + T cells were verified by flow cytometry of peripheral blood mononuclear cells. Twelve weeks later, mice were infected with 50 p.f.u. WSN-SIY virus and 30 dpi SIY-specific CD8 + T cells in various tissues were identified by H-2K b DimerX (BD Biosciences) loaded with SIY peptide plus anti-CD8 by flow cytometry. Gene perturbations and quantitative PCR To perturb the network, selected TFs were overexpressed in CD8 + 2C T cells by retrovirus transduction as described above. Transduced 2C T cells were cultured in the presence of IL-7 for 24 h and GFP + 2C T cells were purified by sorting (>95% viable by PI staining). Total RNA was extracted from the purified 2C T cells using RNeasy micro kit (Qiagen) according to the manufacturer’s instructions. First strand cDNA was synthesized from 1 μg total RNA using the TaqMan Reverse Transcription Reagents (ABI). Diluted cDNA (2 μl; total 200 μl) were used as template for the quantitative PCR with LightCycler480 SYBR Green and LightCycler480 machine (Roche). For each TF-transduced CD8 + T cells, the transcript levels of 12 TFs were measured by qPCR using gene specific primers ( Supplementary Table S5 ). To measure the transcript level of TFs in naive, effector and memory CD8 + T cells, naive 2C T cells were adoptively transferred into B6 mice followed with WSN-SIY virus infection, effector and memory 2C T cells were sorted from spleen 7 dpi and 30 dpi, respectively. Total RNA was isolated from naive, effector and memory 2C T cells and used for quantification of the transcript level of each TF by PCR. ChIP and ChIP-PCR A Millipore ChIP kit was used for chromatin immunoprecipitation. DNA–protein complexes were crosslinked with formaldehyde at a final concentration of 1%, sheared by sonication to 800–1,000 bp, followed by precipitation with nonspecific goat anti-IgG (Sigma) or rabbit anti-IgG (Cell Signaling Technology) or chromatin ChIP-grade anti-Sox4 (C-20, Santa Cruz Biotechnology), anti-Tcf7 (H-118, Santa Cruz Biotechnology) and anti-Eomes (ab23345, Abcam). DNA–protein complex was eluted, and ChIP DNA was purified by PCR purification kit (Qiagen). The promoter regions of the indicated TFs or MSGs were amplified using specific primers ( Supplementary Table S6 ). Primers used to amplify the promoter regions were all within this 1 kb upstream of the transcription-starting site. For ChIP of Bach2 with anti-Bach2 (E-16, Santa Cruz Biotechnology), crosslinked DNA–protein complexes were digested to 400–600 bp by micrococcal nuclease (Cell Signaling Technology). Protein extraction and western blotting Proteins were extracted from transduced 2C T cells with the CelLytic Lysis Reagent (Sigma). Samples containing 20 μg total protein (BCA Protein Assay Kit, Pierce Biotechnology) were resolved on a 10% SDS–PAGE gel and electro-transferred onto a PVDF membrane (Millipore Corporation). The membrane was blocked in 5% ( w / v ) fat-free milk in PBST (PBS containing 0.1% Tween-20). The blot was hybridized overnight with primary antibodies: anti-GAPDH (HRP-conjugated, Cell Signaling Technology, 1:2,000), anti-Sox4 (C-20, Santa Cruz Biotechnology, 1:500), anti-Bach2 (AP10133b, Abgent, 1:500), anti-Id3 (6-1, CalBioreagents, 1:2,500), anti-Blimp-1 (6D3, eBioscience, 1:1,000), anti-Bcl2 (BioLegend, 1:500), anti-Bcl6 (BioLegend, 1:2,000), anti-pFoxO1 (Cell Signaling Technology, 1:1,000), anti-CDK4 (Cell Signaling Technology, 1:1,000), anti-CDK6 (Cell Signaling Technology, 1:1,000), anti-Rb-p780 (Cell Signaling Technology, 1:1,000), anti-Rb-p795 (Cell Signaling Technology, 1:1,000) and anti-p27kip (Cell Signaling Technology, 1:1,000) according to the recommended dilution in 5% fat-free milk. The blot was washed twice in PBST and then incubated with HRP-conjugated secondary antibody (Cell Signaling Technology: anti-Rabbit, 1:2,000; anti-mouse,1:3,000; Santa Cruz Biotechnology: anti-Rat, 1:2,000; anti-Goat 1:3000) in 5% fat-free milk. The membrane was washed twice in PBST and subjected to protein detection by ECL Plus Western Blotting Detection System (GE Healthcare) before being exposed to a Koda BioMax XAR film. The membrane was stripped and re-blotted with the rabbit anti-mouse HRP-conjugated anti-Gapdh antibody (Cell Signaling Technology) for protein loading control. Statistical analysis Statistical significance was determined with the two-tailed unpaired or paired Student’s t -test. P -values for MRA and promoter enrichment results were calculated with a binomial test. The FDRs were computed with q = p × n / i, ( p = P value, n =total number of tests, i =sorted rank of P- value). How to cite this article: Hu, G. and Chen, J. A genome-wide regulatory network identifies key transcription factors for memory CD8 + T-cell development. Nat. Commun. 4:2830 doi: 10.1038/ncomms3830 (2013).